A broadband and strong visible-light-absorbing photosensitizer boosts hydrogen evolution Developing broadband and strong visible-light-absorbing photosensitizer is highly desired for dramatically improving the utilization of solar energy and boosting artificial photosynthesis. Herein, we develop a facile strategy to co-sensitize Ir-complex with Coumarins and boron dipyrromethene to explore photosensitizer with a broadband covering ca. 50% visible light region (Ir-4). This type of photosensitizer is firstly introduced into water splitting system, exhibiting significantly enhanced performance with over 21 times higher than that of typical Ir(ppy) 2 (bpy) + , and the turnover number towards Ir-4 reaches to 115840, representing the most active sensitizer among reported molecular photocatalytic systems. Experimental and theoretical investigations reveal that the Ir-mediation not only achieves a long-lived boron dipyrromethene-localized triplet state, but also makes an efficient excitation energy transfer from Coumarin to boron dipyrromethene to trigger the electron transfer. These findings provide an insight for developing broadband and strong visible-light-absorbing multicomponent arrays on molecular level for efficient artificial photosynthesis. Sunlight-driven water splitting into hydrogen has been regarded as an attractive strategy to simultaneously address the issues of energy crisis and environmental pollution [1] , [2] , [3] , [4] , [5] , [6] , [7] , [8] , [9] , [10] , [11] . As is well known, the solar spectrum exhibits a wide range from ultraviolet region (UV) to infrared region (IR), especially, the visible region covers >40% of solar spectrum [12] . As a result, developing broadband and strong visible-light-absorbing (BSVLA) photosensitizers (PSs) is highly desired for dramatically improving the utilization of solar energy [13] , [14] , [15] . In this field, major progress has been achieved in developing high-efficient catalysts and catalyst–PS coupling molecular devices for efficient hydrogen evolution [2] , [5] , [7] , [8] , [15] , [16] , [17] , [18] , [19] , [20] , [21] . However, the exploitation of highly active PSs are seriously delayed, although they play a critical role in absorbing solar light and mediating electron transfer among photocatalytic system [5] , [8] , [22] , [23] , [24] . In the past decades, noble metal Ru(II)-, Ir(III)-, Pt(II)-, and Re(I)-based molecular complexes, such as Ru(bpy) 3 2+ , Ir(ppy) 2 (bpy) + , and [Pt(tpy)(arylacetylide)] + (tpy = terpyridine), [16] , [19] - [30] are frequently used as PSs for photocatalytic hydrogen evolution due to their long-lived triplet state ( 3 MLCT), which can supply enough time for electron transfer between different components [13] , [14] , [22] , [25] , [26] , [27] , [28] , [29] , [30] , [31] , [32] , [33] , [34] , [35] , [36] . However, the typical MLCT (metal-to-ligand charge transfer) PSs, such as Ir(ppy) 2 (bpy) + ( Ir-1 ), often suffer from weak visible light absorption ability ( ε < 15,000 M −1 cm −1 ) and narrow visible light absorption range, which severely restricted their photocatalytic activity [13] , [14] , [37] . As is well known, organic dyes, such as boron dipyrromethene dye (Bodipy), Coumarin, and Fluorescein, generally exhibit high molar absorption coefficients (~10 5 M −1 cm −1 ) due to the existence of π–π* transition on irradiation [13] , [14] , [38] . Nevertheless, most of these pure organic chromophores are inactive for photocatalytic hydrogen evolution because of their short-lived excited states (<10 ns) [13] , [31] , [32] , [33] , [34] . Against this background, implanting strongly absorbing chromophores into metal complexes has been regarded as an effective strategy to merge the advantages of metal complexes with 3 MLCT state and organic dyes with π–π* transition [15] , [37] , [39] , [40] . In this field, Bodipy, Rhodamine, and Coumarin were widely used to decorate PtN 2 S 2 and Ir(III) complexes to construct strong visible-light-absorbing PSs [15] , [36] , [39] . However, these mono-chromophore-based PSs usually possess narrow visible light absorption range, resulting in low efficiency for solar energy utilization. Integrating two or more different chromophores into the same complex to construct BSVLA PSs for photocatalytic water splitting are still a great challenging task, as it requires efficient intersystem crossing (ISC) process to attain long-lived triplet state and efficient synergism between different chromophores, as well as suitable redox potentials to acquire supporting thermodynamic driving force. Up to date, several attempts have been devoted to exploring BSVLA PSs; however, few of them are competent to absorb solar light and mediate electron transfer in artificial photosynthetic systems to achieve highly efficient water splitting [41] . Herein a co-modification strategy by decorating Ir-based complex with different antennas is explored to construct BSVLA PSs. The resulting Coumarin and Bodipy co-decorating Ir-based PS ( Ir-4 ) display strong visible-light-absorbing ability in the range of 400–575 nm, covering ca. 50% of visible light region. Ir-4 was first used as a highly efficient PS for boosting hydrogen evolution, which exhibits outstanding performance under both 450 and 525 nm light-emitting diode (LED) irradiation. The turnover number (TON) of Ir-4 can reach to 115,840 under optimized condition, which significantly outperforms those of other PSs, and is >320 times higher than that of Ir-1 , demonstrating that Ir-4 is the most active PS among all the reported molecular systems. It is noteworthy mentioning that the Coumarin antenna in Ir-4 can efficiently convert excitation energy to Bodipy by the tandem processes of ISC and triplet–triplet energy transfer (TTET) via Ir mediation. Synthesis and characterization The principle for the design of Ir-4 PS is to directly attach π core of both Coumarin 6 and Bodipy to heavy atom center of Ir(III), which can efficiently mediate the excitation energy of antennas into long-lived triplet state and broaden the visible-light-harvesting range of PSs [14] . For comparison, Ir-1 , Ir-2 , and Ir-3 were also synthesized (Supplementary Fig. 1 ). Ir-1 – Ir-4 were synthesized via a two-step reaction, with the yields >60% (Supplementary Methods) [37] , [40] , [42] . In a typical process, the ppy and Coumarin 6 were used to coordinate with Ir(III) to obtain Ir(III) intermediates of [Ir(ppy) 2 Cl] 2 and [Ir(Coumarin 6) 2 Cl] 2 , respectively. Then the [Ir(ppy) 2 Cl] 2 dimer reacts with bpy and bpy−≡−Bodipy to produce Ir-1 and Ir-3 , respectively. Ir-2 and Ir-4 were prepared by a similar method with that of Ir-3 except using [Ir(Coumarin 6) 2 Cl] 2 to replace [Ir(ppy) 2 Cl] 2 (Supplementary Fig. 1 ). For Ir-4 , the cyclometalated complexing and π-conjugation effect made both Coumarin 6 and Bodipy units closely surround Ir(III) center to maximize the heavy atom effect. All these complexes were well defined and characterized (Fig. 1 , Supplementary Figs. 2 – 15 ), and the structure of Ir-4 was further confirmed by 13 C nuclear magnetic resonance (NMR) (Supplementary Fig. 16 ). Fig. 1 Molecular structures and absorption spectra of photosensitizers. a Molecular structures and ultraviolet−visible absorption spectra of b Ir-1 , c Ir-2 , d Ir-3 , and e Ir-4 in CH 3 CN (5 μM) Full size image Photocatalytic hydrogen evolution To enable better utilization of solar light, exploratory research using BSVLA complex as PS was explored by introducing Coumarin-Ir-Bodipy ( Ir-4 ) into hydrogen evolution system (Fig. 2 , Supplementary Figs. 17 – 21 , and Supplementary Tables 1 and 2 ). Photocatalytic activity of Ir-1 – Ir-4 -containing systems was evaluated in CH 3 CN/H 2 O (v/v = 9/1) with [Co III (dmgH) 2 (py)Cl] ( C-1 ) as catalyst and DMT as sacrificial electron donor (Supplementary Fig. 2 ). As shown in Fig. 2a , ca. 32 μmol H 2 was evaluated from Ir-4 -containing system in 12 h, which was significantly enhanced compared to that of Ir-1 , >21 times higher than that of Ir-1 -containing system. Notably, TON of Ir-4 can reach as high as 115,840 under optimized condition, which represents the most efficient sensitizer among all the reported molecular systems (Supplementary Fig. 19 ) [16] , [43] . Under this condition, the photocatalytic activities of Ir-1 – Ir-3 -containing systems were also investigated, showing the TONs of 361, 22,560, and 8270, respectively. The TON of Ir-4 is >320 times higher than that of Ir-1 , demonstrating that Ir-4 is indeed a state-of-the-art PS. Furthermore, when the concentration of Ir-4 was increased from 1.25 to 30 μM, the yield of hydrogen evolution increased from 32.1 to 120.7 μmol under the irradiation of 175 W Xenon with a 420-nm filter (Fig. 2b ). Fig. 2 Photocatalytic hydrogen evolution. Photocatalytic hydrogen evolution with irradiation of a Xe lamp ( λ > 420 nm, 175 W), b Xe lamp ( λ > 420 nm, 175 W) for different concentrations of Ir-4 , c 525 nm and d 450 nm light-emitting diode with light intensity of 100 mW cm −2 . 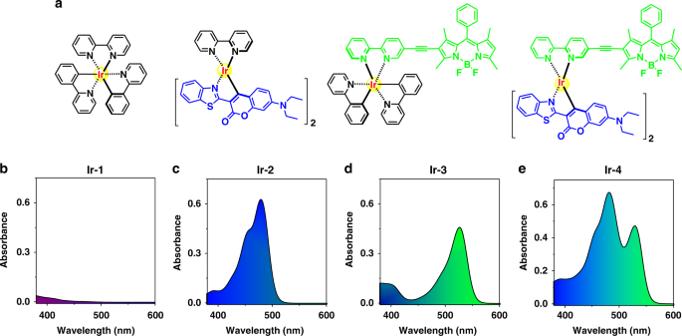Fig. 1 Molecular structures and absorption spectra of photosensitizers.aMolecular structures and ultraviolet−visible absorption spectra ofb Ir-1,c Ir-2,d Ir-3, ande Ir-4in CH3CN (5 μM) Conditions: catalyst (50.0 μM), PS (1.25 μM) and DMT (0.01 M) in CH 3 CN/H 2 O (v/v = 9/1) Full size image Importantly, photocatalytic activity of Ir-4 is almost the sum of Ir-2 and Ir-3 , indicating efficient transfer of excitation energy from Coumarin to Bodipy in Ir-4 (Supplementary Table 1 ). 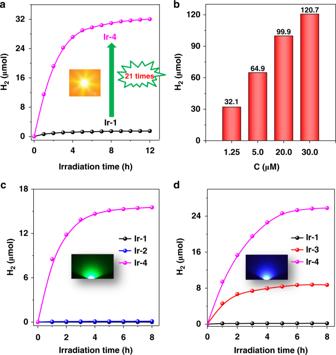Fig. 2 Photocatalytic hydrogen evolution. Photocatalytic hydrogen evolution with irradiation ofaXe lamp (λ> 420 nm, 175 W),bXe lamp (λ> 420 nm, 175 W) for different concentrations ofIr-4,c525 nm andd450 nm light-emitting diode with light intensity of 100 mW cm−2. Conditions: catalyst (50.0 μM), PS (1.25 μM) andDMT(0.01 M) in CH3CN/H2O (v/v = 9/1) Further, isolated Coumarin 6 and Bodipy ligands were simultaneously introduced into the photocatalytic system of Ir-1 with the ratio of Coumarin 6, Bodipy, and Ir-1 same to that in the formula of Ir-4 , and photocatalytic study reveals that the activity of the mixture is similar to that of Ir-1 , far lower than that of Ir-4 -containing system (Supplementary Table 2 , Entry 9). These results indicate that Coumarin 6 and Bodipy cannot sensitize Ir-1 due to the far distance between the antenna molecules and Ir-1 in the physical mixture. Also, in the absence of Ir-1 , trace amount of H 2 was produced with Coumarin 6 and Bodipy ligands as the PSs, revealing that the Ir mediation can enable inactive pigments as efficient light-harvesting molecules for water splitting. In addition, no or little hydrogen was detected in the absence of light, C-1 , DMT , PS, and H 2 O, manifesting that all above factors were indispensable for efficient hydrogen evolution (Supplementary Table 2 ). All the above results indicate that the BSVLA ability of Ir-4 , resulting from closely decorating Ir(III) center with Coumarin 6 and Bodipy, greatly contributes to boosting its photocatalytic activity. In order to further highlight the advantage of BSVLA Ir-4 , photocatalytic experiments were carried out with 450 and 525 nm LED (corresponding to the absorption of Coumarin 6 and Bodipy, respectively) as monochromatic light source, respectively (Fig. 2c, d ). The photocatalytic activity of Ir-4 was obviously superior to that of Ir-3 and Ir-2 upon excitation at 450 and 525 nm, respectively, indicating that Ir-4 was potential for breaking the limitation of narrow absorption band of mono-chromophore PSs. Ir-1 gives an extremely weak activity in hydrogen evolution upon LED irradiation at either 450 or 525 nm due to its poor visible-light-harvesting ability [42] . In addition, the apparent quantum yield of Ir-4 was estimated to be 37.7% at 475 nm and 25.1% at 520 nm based on the incident photons [44] , [45] . In order to ascertain the actual source of protons, the photocatalytic products in the presence of H 2 O and D 2 O were both studied by using mass spectrometry (MS) analysis (Supplementary Fig. 21 ) [46] , [47] . H 2 as the sole gaseous product was detected by MS in the mixed solvents of H 2 O and CH 3 CN, and D 2 became the major product when replacing H 2 O with D 2 O. In addition, only trace amount of hydrogen can be detected with pure CH 3 CN as solvent in the absence of H 2 O. These results confirm the H 2 O as the source of protons and exclude the dehydrogenation of DMT or CH 3 CN. Systematic investigation of steady spectra, transient spectra, electrochemistry, and density functional theory (DFT) calculation reveal that the improved activity of Ir-4 can be ascribed to the comprehensive factors, such as strong visible-light-harvesting ability, efficient electron transfer, suitable redox potential, and excited state type with long excited state lifetime. Steady absorption and emission spectra To decipher the intrinsic properties of PSs and electron transfer process between different components, steady spectra of PS alone and PS with C-1 or DMT were performed, respectively. UV-vis absorption spectra of Ir-2 and Ir-3 show strong absorption band around 475 and 530 nm, corresponding to the absorption of Coumarin 6 and Bodipy, respectively (Supplementary Fig. 22 ) [37] , [40] , [42] . Ir-4 shows a broad absorption band between 400 and 575 nm, which is almost superposition of the absorption of Ir-2 and Ir-3 (Supplementary Fig. 22a ). This result indicates no electronic interaction between Bodipy and Coumarin 6 in Ir-4 under the ground state. Furthermore, UV-vis absorption spectra of PS alone, PS with C-1 , PS with DMT , and PS with both C-1 and DMT were all studied in detail (Supplementary Fig. 23 ). Related results show that the absorption spectra of Ir-2 – Ir-4 stay almost unchanged before and after adding DMT , C-1 , or DMT and C-1 , indicating no electronic interaction between PSs in the ground state and DMT (or C-1 ). The emission spectra of Ir-1 – Ir-4 were studied under different atmospheres (Fig. 3a–d and Supplementary Figs. 24 – 25 ). In nitrogen, Ir-1 gave an emission peak around 585 nm, and Ir-2 – Ir-4 show dual emission peaks at 507/586, 556/745, and 506/557 nm, respectively. The peaks at 585 nm for Ir-1 , 586 nm for Ir-2 , and 745 nm for Ir-3 became weaker or disappeared in the air, indicating that these peaks could be attributed to phosphorescence (PL) originating from triplet excited states (TESs) of these complexes [13] , [40] , [42] . No significant change for other peaks under different atmospheres manifested that these peaks should be the residual fluorescence (FL) of chromophores, derived from their singlet excited states (SESs). These results were further verified by emission lifetime (Fig. 3e and Supplementary Fig. 26 ). No or weak PL was observed for Ir-4 and Ir-3 due to the presence of Bodipy-localized 3 IL state [42] , [48] . Isolated Coumarin 6 and Bodipy usually showed strong FL; however, their FL was completely quenched in Ir-2 – Ir-4 owing to an efficient ISC process from SES to TES (Supplementary Fig. 24 ). Fig. 3 Emission quenching. a Ir-3 with DMT ( λ ex = 510 nm), b zoom in the range between 725 and 800 nm, c Stern–Volmer plot of fluorescence and phosphorescence by DMT ; d the emission of Ir-3 under nitrogen and air atmosphere; e emission lifetime of Ir-3 at 556 nm, λ ex = 510 nm, and f photophysical process of Ir-3 upon light excitation. ET electron transfer, GS ground state, ISC intersystem crossing. c PS = 5.0 μM Full size image In this process, the emission quenching experiments of Ir(III) complexes by DMT and C-1 were carried out to study the electron transfer efficiency (Fig. 3b, c and Supplementary Figs. 27 – 29 ). The efficiency of FL quenching of Ir-2 and Ir-3 by DMT and C-1 is far lower than that of PL quenching, indicating that long-lived triplet state is more beneficial to electron transfer than short-lived singlet state [22] , [38] . Thus the initial step of electron transfer process should be dominated by triplet states of Ir(III) complexes. The efficiency of electron transfer can be determined by PL quenching experiments. 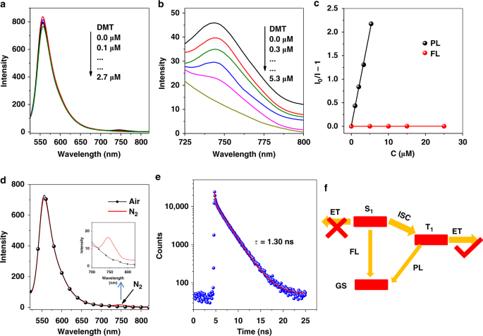Fig. 3 Emission quenching.a Ir-3withDMT(λex= 510 nm),bzoom in the range between 725 and 800 nm,cStern–Volmer plot of fluorescence and phosphorescence byDMT;dthe emission ofIr-3under nitrogen and air atmosphere;eemission lifetime ofIr-3at 556 nm,λex= 510 nm, andfphotophysical process ofIr-3upon light excitation. ET electron transfer, GS ground state, ISC intersystem crossing.cPS= 5.0 μM The K sv quenching constants of PSs quenched by DMT were in the order of Ir-3 (407,200 M − 1 ) > Ir-1 (3607 M −1 ) > Ir-2 (224 M −1 ), proportional to their triplet lifetimes (Supplementary Table 3 ). As shown in Fig. 3f , upon 510 nm excitation, the SES of Ir-3 was populated and then afforded a triplet state via ISC process. As result, Ir-3 can emit FL and PL simultaneously, providing the first molecular platform that can directly evaluate electron transfer ability between singlet state and triplet state in same one molecule with dual emission. For DMT quenching, the quenching constant of PL can reach to ca. 4.1 × 10 5 M −1 , >7000 times higher than that of the FL quenching (56.2 M −1 ). A series of experiments reveal that the electron transfer efficiency from long-lived triplet state significantly outperforms that from short-lived excited state. Electrochemical study In order to assess the thermodynamic feasibility of electron transfer, redox potentials of Ir-1 – Ir-4 , DMT , and C-1 were determined in CH 3 CN/H 2 O (v/v = 9/1) (Fig. 4 , Supplementary Figs. 30 – 31 , Supplementary Tables 1 and 4 ) by the cyclic voltammetry (CV) (Supplementary Methods). Ir-1 gave an oxidation potential at 1.31 V and a reduction potential at −1.37 V, corresponding to the redox processes from Ir 3+ to Ir 4+ and bpy 0 to bpy −1 , respectively. For Ir-2 containing two Coumarin 6 units, three reduction potentials at −1.19, −1.45, and −1.66 V can be attributed to Coumarin 6 0/−1 , Coumarin 6 –1/−2 , and bpy 0/−1 , respectively. The first reduction potential of Ir-3 was determined as −0.94 V, less negative than that of Ir-1 and Ir-2 as the existence of reduction process from Bodipy 0 to Bodipy −1 . Ir-4 also shows three reduction potentials at −0.94, −1.12, and −1.46 V, respectively. The first reduction potential of Ir-4 was same as that of Ir-3 , as well as the second and third reduction potentials of Ir-4 were very close to the first two reduction potentials of Ir-2 , indicating that the reduction potentials of Ir-4 correspond to the redox process of Coumarin 6 and Bodipy units, respectively (Table 1 ). Accordingly, there was hardly any electron interaction between Coumarin and Bodipy ligands in Ir-4 under the ground state, which well matched the results of absorption spectra. Additionally, the oxidation potential of Ir-2 was determined as 1.12 V, less positive than that of Ir-1 and Ir-3 , and Ir-3 possesses of an oxidation potential of 1.28 V, very close to that of Ir-1 . These results manifested that Coumarin had a more significant effect on the oxidation potential of Ir-based complexes in comparison with the Bodipy unit. As a result, it is reasonable that the oxidation potential of Ir-4 (1.19 V) was close to that of Ir-2 . Fig. 4 Electrochemical study. Cyclic voltammograms of a Ir-1 , b Ir-2 , c Ir-3 , and d Ir-4 were determined in deaerated CH 3 CN/H 2 O (v/v, 9/1) solution, containing 0.5 mM photosensitizer, ferrocene, and 0.10 M Bu 4 NPF 6 as the supporting electrolyte, with a scan rate of 0.05 V/s −1 and a negative initial scan direction. Glassy carbon electrode, Ag/AgNO 3 , and Pt silk were used as the working electrode, reference electrode, and counter electrode, respectively Full size image Table 1 Redox potentials of Ir-1–Ir-4 and the ΔG CS for intermolecular electron transfer Full size table CV of C-1 was also performed in deaerated CH 3 CN and CH 3 CN/H 2 O (v/v, 9/1) solution to uncover its catalytic mechanism (Supplementary Fig. 32 ) [49] , [50] , [51] . The redox process of Co 2+ /Co + at −1.09 V (vs. saturated calomel electrode (SCE)) remained reversible in water-containing system, indicating that it is impossible to carry out catalytic water splitting at this potential [49] . Interestingly, a large catalytic current emerged at around −1.48 V (vs. SCE) corresponding to the redox process of Co + /Co 0 , which could be attributed to the proton reduction process in the presence of Co(0) species [51] . 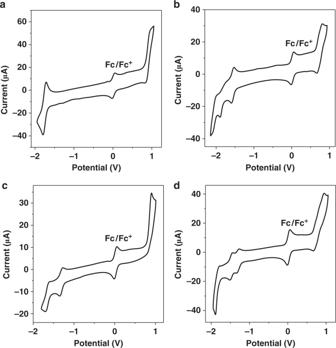Fig. 4 Electrochemical study. Cyclic voltammograms ofa Ir-1,b Ir-2,c Ir-3, andd Ir-4were determined in deaerated CH3CN/H2O (v/v, 9/1) solution, containing 0.5 mM photosensitizer, ferrocene, and 0.10 M Bu4NPF6as the supporting electrolyte, with a scan rate of 0.05 V/s−1and a negative initial scan direction. Glassy carbon electrode, Ag/AgNO3, and Pt silk were used as the working electrode, reference electrode, and counter electrode, respectively Considering that the possibility of electron transfer from reduced PSs to Co + was thermodynamically ruled out, we tentatively proposed that the disproportionation of Co + into Co 2+ and Co 0 was a possible pathway in this photocatalytic system [52] . 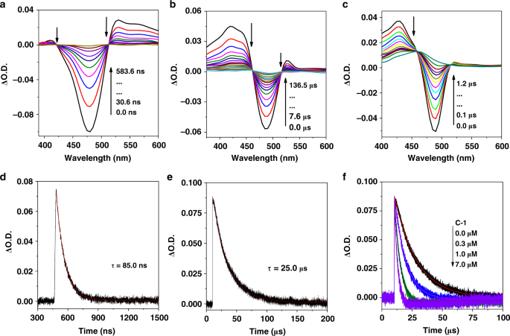Fig. 5 Nanosecond transient absorption spectra of Ir-2.a Ir-2,b Ir-2with 40 mM ofDMT,creducedIr-2with 0.2 mM ofC-1;dthe decay ofIr-2at 468 nm,ekinetic traces of reducedIr-2followed at 500 nm,fkinetic traces of reducedIr-2with different concentration ofC-1followed at 500 nm. These spectra were recorded in CH3CN after pulsed excitation at 355 nm under N2 Further, electrolysis experiment of C - 1- containing system was performed to confirm this view, where H 2 was indeed detected at −1.09 V (vs. SCE, corresponding to Co(II)/Co(I)), indicating the formation of Co 0 species during this electrolysis process (Supplementary Table 5 ). The Gibbs free energy changes ( ΔG CS ) of electron transfer from DMT to excited PSs, from excited PS to C-1 , and from reduced PSs to C-1 were figured out by Weller equation (Supplementary Eqs. 1 – 3 ) [53] , [54] , [55] . The negative values of ΔG CS for all the reduction processes indicate the thermodynamic feasible for relevant electron transfer. For the oxidation process, the electron transfer from excited Ir-3 to Co 2+ and excited Ir-4 to Co 2+ were restricted owing to the positive values of ΔG CS (0.40 for Ir-3 and 0.31 for Ir-4 ), which thermodynamically ruled out the possibility of oxidation mechanism. Therefore, photocatalytic route of these photocatalytic systems can be determined as the reduction mechanism according to the electrochemical results. The absolute values of ΔG CS of excited Ir-1 / DMT (0.44) and Ir-2 / DMT (0.52), as well as reduced Ir-1 /Co 2+ (0.45) and reduced Ir-2 /Co 2+ (0.27), were much larger than those of related processes of Ir-3 and Ir-4 . These results demonstrated much larger driven forces from DMT to excited Ir-1 and from reduced Ir-1 to C-1 in comparison with those of Ir-3 - and Ir-4 -containing systems. However, Ir-1 exhibits the lowest activity among these four compounds, and this can be largely attributed to its poor visible-light-harvesting ability. Further, Ir-4 containing three additional antennas exhibits the best photocatalytic performance among Ir-1 – Ir-4 , although it shows a humble driven force for electron transfer. Hence, it can be proposed that the BSVLA ability and long-lived excited state of Ir-4 plays an important role in dramatically improving its photocatalytic performance. As a result, Ir-4 was determined to be the most efficient PSs among Ir-1 – Ir-4 for hydrogen evolution with the TON reaching 115,840, representing the most active sensitizer among all the reported molecular photocatalytic systems. Transient absorption spectra Nanosecond transient absorption spectra were investigated in degassing CH 3 CN to shed light on the photocatalytic process (Figs. 5 and 6 and Supplementary Figs. 33 – 35 ). Upon excitation at 355 nm, Ir-1 showed two positive absorption bands around 380 and 490 nm, similar to previous report, and its lifetime was determined as 307 ns (Supplementary Fig. 33 ) [42] . By addition of DMT , a long-lived species of reduced Ir-1 was obtained with a decay of 63 μs (Supplementary Fig. 33e ). In the presence of C-1 , the decay of reduced Ir-1 was significantly faster, supporting an extra electron transfer pathway from reduced Ir-1 to C-1 . For Ir-2 , a strong bleaching peak around 475 nm was observed upon pulsed laser excitation, corresponding to its ground state absorption (Fig. 5a ). The triplet state of Ir-2 was localized on Coumarin 6 with a triplet state lifetime of 85 ns (Fig. 5d ). After adding DMT , the bleaching peak shows a redshift from 475 to 487 nm, and two new positive absorption bands between 380/460 and 525 nm/550 nm appeared, indicating the formation of new transient species with a long-lived decay at 500 nm (25.0 μs) (Fig. 5b, e ). This new species can be identified as the reduced state of Ir-2 , further supported by PL quenching experiments. The reduced Ir-2 with C-1 shows a faster decay to baseline than that of reduced Ir-2 alone, manifesting an efficient electron transfer from reduced Ir-2 to C-1 (Fig. 5c, f ). As a result, the photocatalytic process of Ir-1 - and Ir-2 -containing systems is mainly dominated by reduction mechanism. Fig. 5 Nanosecond transient absorption spectra of Ir-2. a Ir-2 , b Ir-2 with 40 mM of DMT , c reduced Ir-2 with 0.2 mM of C-1 ; d the decay of Ir-2 at 468 nm, e kinetic traces of reduced Ir-2 followed at 500 nm, f kinetic traces of reduced Ir-2 with different concentration of C-1 followed at 500 nm. These spectra were recorded in CH 3 CN after pulsed excitation at 355 nm under N 2 Full size image Fig. 6 Nanosecond transient absorption spectra of Ir-4. a Ir-4 , b Ir-4 in the presence of 40 mM of DMT , c reduced Ir-4 in the presence of 0.2 mM of C-1 , d the decay of Ir-4 at 517 nm, e kinetic traces of the reduced Ir-4 followed at 525 nm, f kinetic traces of reduced Ir-4 with different concentration of C-1 followed at 525 nm. These spectra were recorded in CH 3 CN after pulsed excitation at 532 nm under N 2 Full size image Compared to Ir-2 , transient absorption spectrum of Ir-3 exhibits a strong bleaching peak at 525 nm upon pulsed laser excitation at 532 nm, which well matched with the ground state absorption of Bodipy (Supplementary Fig. 34 ) [42] . Hence, triplet state of Ir-3 was populated on the Bodipy part, further confirmed by its long-lived excited state ( τ T = 101 μs) (Supplementary Fig. 34a, d ). In the presence of DMT , both the positive peak around 430 nm and the bleaching peak at 523 nm obviously decreased, meanwhile, a new peak at 580 nm rose, indicating the formation of a new species (Supplementary Fig. 34b ). The lifetime of this species was up to 113 μs, even longer than that of Ir-3 alone (Supplementary Fig. 34e ). As is well known, the triplet state of Ir-3 could be efficiently quenched by DMT through an electron transfer process. Accordingly, we proposed the new species as the reduced Ir-3 . Similar to Ir-2- containing system, transient spectra confirmed that the reduced Ir-3 can be efficiently oxidized by C-1 (Supplementary Fig. 34c, f ). As a result, reduction mechanism for Ir-3 -containing system should be a dominant electron transfer process. The photophysical processes of Ir-4 with multiple chromophores should be more complex in comparison with that of Ir-2 or Ir-3 (Fig. 6 ). Upon excitation at either 532 or 470 nm, the transient spectrum of Ir-4 was similar to that of Ir-3 , indicating that the excited state of Ir-4 was also distributed on the Bodipy part (Fig. 6a, d ). This can be ascribed to the lower triplet energy level of Bodipy than that of Coumarin antenna. Notably, transient spectra of Ir-4 remained unchanged upon exciting Coumarin and Bodipy ligands, signifying that the Coumarin antenna could deliver fast excitation energy to Bodipy (>10 8 s −1 ) (Supplementary Fig. 35 ). After adding DMT , a long-lived reduced state of Ir-4 (88.7 μs) was obtained, verified by the similar method of Ir-3 (Fig. 6b, e ). In the presence of C-1 , the transient spectra of reduced Ir-4 returned more quickly to the baseline, and the decay at 525 nm became more faster by increasing the concentration of C-1 with a second-order rate constant of 8.1 × 10 10 M −1 s −1 , revealing an efficient electron transfer from reduced Ir-4 to C-1 (Fig. 6c, f ). Consequently, the reduction quenching pathway should be a dominant process for Ir-4 -containing system. To further confirm the presence of reduced species of the PSs, spectroelectrochemical (SEC) experiments were performed in the Ar atmosphere [43] . As shown in Supplementary Fig. 36 , the transient absorption spectra of Ir-1 – Ir-4 with DMT matched well with the absorption of reduced PSs but were different from that of the oxidized ones (Supplementary Fig. 37 ). Thus the transient absorption spectra of Ir-1 – Ir-4 with DMT could be assigned to the absorption of reduced PSs. Femtosecond transient absorption spectroscopy of Ir-4 was carried out to clarify its intramolecular energy transfer process (Supplementary Fig. 38 ) [56] , [57] , [58] . Upon selective excitation at 438 nm (corresponding to Coumarin ligand), both the bleaching peak at 481 nm and excited state absorption band beyond 600 nm for the triplet state of Coumarin 6 decreased, accompanied by the enhancement of the bleach signal around 528 nm and excited state absorption band at 440 nm of the triplet state of Bodipy (Figs. 5a and 6a ). Therefore, this process can be attributed to intramolecular TTET and its rate constant was determined to be k TTET = 4.3 × 10 10 s −1 by monitoring the increase of bleaching band at 528 nm. It should be noted that no ISC process can be observed with this femtosecond transient absorption spectroscopy, indicating an ultrafast ISC process. This can be ascribed to the fact that the cyclometalated complexing approach made Coumarin 6 closely surround Ir(III) center to maximize the heavy atom effect. Both Ir-3 and Ir-4 show long-lived triplet state with the lifetime of 101 and 89 μs, respectively. By contrast, the triplet lifetimes of Ir-1 and Ir-2 were merely 307 and 85 ns, respectively, which is to the disadvantage of the electron transfer between different components. In addition, all these complexes show a long-lived reduced state (63.0, 25.0, 113.0, and 88.7 μs for Ir-1 , Ir-2 , Ir-3 , and Ir-4 , respectively), and the second-order rate constants from reduced Ir-1 – Ir-4 by C-1 were determined as 2.0 × 10 10 , 1.7 × 10 11 , 2.8 × 10 10 , and 8.1 × 10 10 M −1 s −1 , respectively, which were proximate to the diffusion-controlled limits (Supplementary Fig. 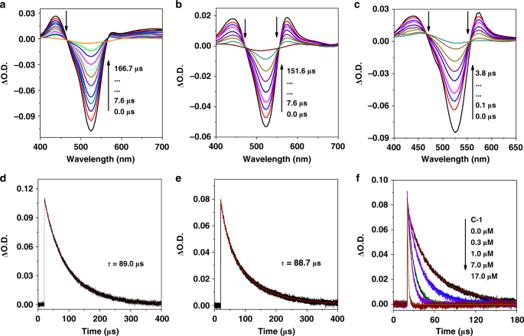Fig. 6 Nanosecond transient absorption spectra of Ir-4.a Ir-4,b Ir-4in the presence of 40 mM ofDMT,creducedIr-4in the presence of 0.2 mM ofC-1,dthe decay ofIr-4at 517 nm,ekinetic traces of the reducedIr-4followed at 525 nm,fkinetic traces of reducedIr-4with different concentration ofC-1followed at 525 nm. These spectra were recorded in CH3CN after pulsed excitation at 532 nm under N2 39 and Supplementary Table 6 ) [59] . These results indicate that the long-lived triplet state for Ir-3 and Ir-4 can supply enough time for efficient electron transfer between PS and other components in these three component systems and Ir-4 possessed BSVLA ability, long-lived triplet state, and long-lived reduced state, highlighting that Ir-4 could act as an efficient PS for promoting hydrogen evolution. DFT calculations on Ir-1–Ir-4 DFT calculation represents a powerful method to unveil the property of excited states of PSs. Herein the population of excited states and photophysical processes of Ir-4 were both evaluated by time-dependent DFT (TDDFT) method (Figs. 7 and 8 ). For Ir-1 , the spin density was localized on ppy and Ir center, indicating the presence of both 3 MLCT and 3 IL states, which were also localized on bpy, Coumarin, and Ir center in Ir-2 . The distribution of spin density can rationalize the short-lived TES of Ir-1 and Ir-2 (Fig. 5d ). The spin density of both Ir-3 and Ir-4 mainly distributed on Bodipy part, the Ir(III) center, bpy, and Coumarin ligands made little contribution, indicating that their lowest-lying TESs could be attributed to Bodipy-localized 3 IL state. Notably, these results are well consistent with the results of PL and transient absorption spectra. Fig. 7 Spin density surfaces. Spin density surfaces of Ir-1 – Ir-4 were calculated at B3LYP/6–31G/genecp/LanL2DZ level with Gaussian 09 Full size image Fig. 8 Selected frontier molecular orbitals involved in the excitation and singlet excited state/triplet excited state (TES) of Ir-4. VR stands for vibrational relaxation. The left column is ultraviolet–visible absorption (based on ground state geometry), the middle column is the fluorescence emission (based on S 1 state geometry), and the right column is the TES (based on ground state geometry). For clarity, only selected excited states are presented Full size image In order to track the evolution of intramolecular photophysical processes of Ir-4 , UV-vis absorption, FL, and TESs were evaluated based on optimized ground-state geometry with TDDFT method (Fig. 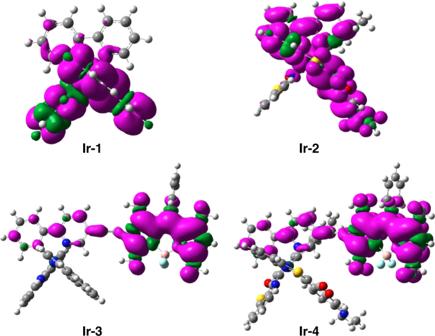Fig. 7 Spin density surfaces. Spin density surfaces ofIr-1–Ir-4were calculated at B3LYP/6–31G/genecp/LanL2DZ level with Gaussian 09 8 and Supplementary Table 7 ). For UV-vis absorption, two major transitions (S 0 → S 3 and S 0 → S 16 ), judged by the oscillator strength, were located at 589 and 418 nm and the corresponding molecular orbitals were distributed on Bodipy and Coumarin ligands in Ir-4 , respectively. These results matched well with experimental results of absorption spectra. The calculated results reveal that the SESs of S 1 and S 2 were both the charge transfer states as their negligible oscillator strength. The transition of S 3 → S 0 corresponded to conversion of electronic cloud distribution in Bodipy, which was in line with the emission spectra of Ir-4 . As the heavy atom effect of Ir, the SES of Ir-4 can efficiently transform into triplet state via an ISC process. The T 1 state was localized on the Bodipy unit, which fully agreed with transient absorption spectra and spin density surfaces of Ir-4 . In addition, T 5 and T 6 states were populated on two Coumarin ligands and they were degenerate due to the similar energy level of triplet state (2.12 eV for T 5 and 2.16 eV for T 6 ). As a result, the whole photophysical processes of Ir-4 were rationalized by DFT/TDDFT calculations (Fig. 8 ), confirming the efficient energy transfer from Coumarin to Bodipy and the population of the long-lived Bodipy-localized 3 IL state, which can efficiently trigger the electron transfer to afford redox reactions. In a word, the photocatalytic cycle of Ir-1 – Ir-4 -containing systems proceeded via a reductive route. For Ir-4 -containing system, both Bodipy and Coumarin ligands can be excited by visible light, and subsequently electron transfer proceeded by two different pathways. As shown in Fig. 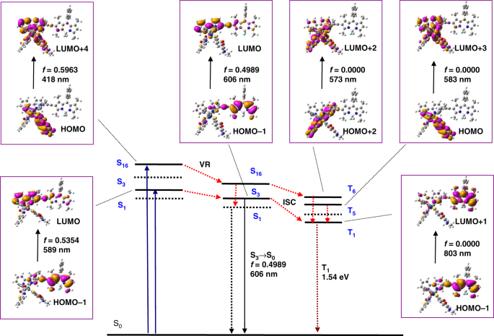Fig. 8 Selected frontier molecular orbitals involved in the excitation and singlet excited state/triplet excited state (TES) of Ir-4. VR stands for vibrational relaxation. The left column is ultraviolet–visible absorption (based on ground state geometry), the middle column is the fluorescence emission (based on S1state geometry), and the right column is the TES (based on ground state geometry). For clarity, only selected excited states are presented 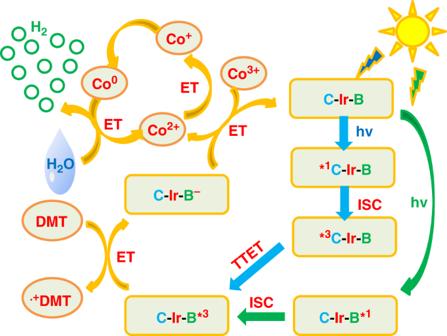Fig. 9 Proposed photochemical process for hydrogen evolution with Ir-4 (C-Ir-B). Ir is the coordination center, C is Coumarin, B is Bodipy, ET is electron transfer, ISC is intersystem crossing, TTET stands for triplet-triplet energy transfer 9 , upon exciting the Bodipy part, the triplet state of Ir-4 was populated on Bodipy by a photochemical process of [C-Ir-B] → 1 [C-Ir-B*] → 3 [C-Ir-B*]. When exciting Coumarin unit, a more complex photophysical process was revealed as follows: [C-Ir-B] → 1 [*C-Ir-B*] → 3 [*C-Ir-B] → 3 [C-Ir-B*]. Hence, Bodipy-localized triplet state of Ir-4 could accept electron from DMT to generate the reduced Ir-4 , which further efficiently delivered electrons to C-1 to produce Co(I). However, the possibility of electron transfer from reduced Ir-4 to Co(I) was thermodynamically ruled out. Thus the formation of Co(0) species could be attributed to the disproportionation of Co(I) into Co(II) and Co(0) [52] . Finally, the protons were reduced to hydrogen by reduced C-1 . As a result, Ir-4 with multichromophores showed dual excitation channels, which can promote solar energy conversion and the subsequent photocatalytic water splitting. Fig. 9 Proposed photochemical process for hydrogen evolution with Ir-4 (C-Ir-B). Ir is the coordination center, C is Coumarin, B is Bodipy, ET is electron transfer, ISC is intersystem crossing, TTET stands for triplet-triplet energy transfer Full size image In conclusion, Bodipy and Coumarin ligands with strong visible light absorption bands in different regions were delicately integrated into a Ir(III) complex to dramatically improve the utilization of solar energy. Ir-4 exhibits a BSVLA range from 400 nm to 575 nm that can cover ca. 50% of visible light region. Systematic experimental investigations and DFT calculations thoroughly rationalize the photophysical process, where Ir mediation made an efficient excitation energy transfer from Coumarin to Bodipy to trigger the redox reactions. In this process, the Coumarin in Ir-4 can absorb the light and efficiently convert excitation energy into Bodipy-localized triplet state by the cascade processes of ISC and intramolecular TTET, which can further promote electron transfer process from DMT to excited Ir-4 and subsequently photocatalytic hydrogen evolution. The BSVLA PS was first introduced into water splitting system, exhibiting significantly enhanced photocatalytic performance >320 times higher than that of typical Ir-1 , and the TON towards Ir-4 reaches to 115,840, representing the most active sensitizer among all the molecular systems. Much enhanced photocatalytic activity of Ir-4 was mainly attributed to its BSVLA ability, long-lived excited state, and delicate synergistic effect between different components. This work paves the way to develop BSVLA multicomponent array on molecular level for efficient solar light conversion and boosting artificial photosynthesis. Materials and methods All the reactions were performed in argon unless otherwise mentioned. All the solvents were of analytical grade and distilled before use. IrCl 3 •3H 2 O and Coumarin 6 was purchased from Sigma-Aldrich. 2-Phenylpyridine, NH 4 PF 6 , and N -iodosuccinimide were purchased from HEOWNS. Triphenylphosphine, dichlorobis(triphenyl-phosphine)palladium(II), CuI, and 2,2'-bipyridine were purchased from Adamas-beta. Chromatographic-grade acetonitrile was purchased from Adamas Reagent. The synthetic scheme of Ir-1 – Ir-4 is presented in Supplementary Fig. 1 . The synthetic intermediates and target complexes were evidenced by 1 H NMR and mass spectroscopy. Instruments The amount of the hydrogen product was analyzed by gas chromatography (Shimadzu GC-2014+AT 230C, TDX-01 column, TCD, argon carrier). UV-vis absorption spectra were recorded on a LAMBDA750 UV-vis spectrophotometer. FL spectra were taken on Hitachi F4600 spectrofluorometer. Transient absorption spectra were measured on the LP980 laser flash photolysis instrument (Edinburgh, UK). FL lifetime was performed by time-resolved confocal FL instrument (MicroTime 200, PicoQuant, Berlin, Germany). Photocatalytic experiments were conducted with 450 and 525 nm LED light (Zolix, MLED4) and 175 W Xenon lamp (LX-175, PEILC, Japan) with 420 nm filter. Electrochemical measurements were carried out on a CHI 760E electrochemical workstation at room temperature. Photocatalytic hydrogen production Photocatalytic hydrogen evolution was conducted under 1 atm of Ar at 25 °C in 16 mL reactor containing PS (1.25 μM), C-1 (50 μM), DMT (10 mM), 0.5 mL H 2 O, and 4.5 mL CH 3 CN. The mixture was continuously stirred and irradiated under a Xe lamp ( λ > 420 nm, 122 mW cm −2 ). Spectrum measurement All the solvents were chromatographically pure for spectra measurement, and all the measurements were performed under an argon atmosphere unless otherwise stated. For guaranteeing the accuracy of the test outcomes, Ru(bpy) 3 2+ served as standard sample to correct the instrument and the method of measurement. Measurement of apparent quantum efficiency (AQE) AQE was measured under the same photocatalytic reaction condition and 175 W Xe lamp fitted with the 475 and 520 nm band-pass filters, and AQE was calculated according to Eq. 1 : 
    AQE = ( number of reacted electrons/number of incident photons) × 100 =
    [ ( number of evolved H_2 molecules× 2 )/number of incident photons] × 100
 (1) The number of incident photons was 2.6 × 10 19 photons h −1 at 475 nm and 2.5 × 10 19 photons h −1 at 520 nm, which was measured by using a calibrated Si photodiode (HAMAMATSUS2281). Isotope tracer experiment The isotope tracer experiment was performed by using D 2 O to replace H 2 O in the photocatalytic H 2 evolution process while all other constituents remained the same. After the photocatalytic reaction, the gaseous product was analyzed with MS (HIDEN ANALYTICAL, HAS-301–144FPL). The background of H 2 was collected from the container containing pure CH 3 CN under 1 atm of Ar. Spectroelectrochemistry SEC experiments were executed in the anhydrous CH 3 CN under nitrogen atmosphere. These measurements were performed using controlled-potential electrolysis (CHI 760E electrochemical workstation) at potentials 50–100 mV more negative than the reduction potential or 50–100 mV more positive than the oxidation potential of complexes Ir-1 – Ir-4 . Electrolyses was carried out on a reticulated Pt electrode with three-dimensional meshes (0.8 × 0.5 × 0.1 cm 3 ). The auxiliary electrode was a Pt wire. The solution in 1 mm path-length cell mainly contained 0.1 mM PS, 0.6 mL CH 3 CN, and 0.1 M [Bu 4 N]PF 6 . The change in absorption due to the reduction or oxidation of the PSs was monitored by the HITACHI optic spectrophotometer (U-3900) for UV−visible experiments equipped with both deuterium (D 2 ) and tungsten iodide (WI) light sources (2J1–1500, 885–1200, HITACHI Optics). Femtosecond transient absorption spectra The pump beam was generated from a regenerative amplified Ti: sapphire laser system from Coherent (800 nm, 100 fs, 6 mJ per pulse, and 1 kHz repetition rate). Output pulse of 800 nm from the regenerative amplifier was split into two parts with a beam splitter. The reflected part was used to pump a TOPAS Optical Parametric Amplifier, which generates a wavelength-tunable laser pulse from 250 nm to 2.5 µm as pump beam. The transmitted 800-nm beam was attenuated with a neutral density filter and focused into a rotating CaF 2 disk to generate a white light continuum from 350 to 800 nm used for probe beam. The probe beam was focused with an Al parabolic reflector onto the sample. After penetrating the sample, the probe beam was collimated to focus into a fiber-coupled spectrometer and detected at a frequency of 1 KHz. The intensity of the pump pulse used in this experiment was controlled by a variable neutral-density filter wheel. The delay between the pump and probe pulses was controlled by a motorized delay stage. The pump pulses were chopped by a synchronized chopper at 500 Hz. The pump pulse was kept in a weak regime where the excitonic annihilation effect can be neglected. DFT calculation The geometries and the spin density surfaces of the complexes ( Ir-1 – Ir-4 ) were performed at the B3LYP/6–31G/LanL2DZ level. There are no imaginary frequencies for all optimized structures of Ir-1 – Ir-4 . The UV-vis absorption, the FL, and the triplet state energy levels were carried out with the TDDFT method. VR stands for vibrational relaxation, indicating the transition from v = x ( x > 0) level of excited state to v = 0 level of excited state (Fig. 8 ). All these calculations were performed with Gaussian 09 program [60] . Other methods Other information about syntheses, characterizations, and cyclic voltammograms of compounds are given in Supplementary Information.